Structure-guided mutational analysis reveals the functional requirements for product specificity of DOT1 enzymes DOT1 enzymes are conserved methyltransferases that catalyse the methylation of lysine 79 on histone H3 (H3K79). Most eukaryotes contain one DOT1 enzyme, whereas African trypanosomes have two homologues, DOT1A and DOT1B, with different enzymatic activities. DOT1A mediates mono- and dimethylation of H3K76, the homologue of H3K79 in other organisms, whereas DOT1B additionally catalyses H3K76 trimethylation. However, it is unclear how these different enzymatic activities are achieved. Here we employ a trypanosomal nucleosome reconstitution system and structure-guided homology modelling to identify critical residues within and outside the catalytic centre that modulate product specificity. Exchange of these residues transfers the product specificity from one enzyme to the other, and reveals the existence of distinct regulatory domains adjacent to the catalytic centre. Our study provides the first evidence that a few crucial residues in DOT1 enzymes are sufficient to catalyse methyl-state-specific reactions. These results might also have far-reaching consequences for the functional understanding of homologous enzymes in higher eukaryotes. In every eukaryotic cell, the nucleosome is the basic repetitive unit of chromatin, which is formed by double-stranded DNA wrapped around a histone octamer composed of two copies of each core histone H2A, H2B, H3 and H4 (refs 1 , 2 , 3 ). Histones are subject to a variety of posttranslational modifications, which influence chromatin structure and function [4] , [5] . Among these modifications, methylation is catalysed by lysine and arginine methyltransferases that transfer a methyl group from the cofactor S -adenosyl- L -methionine (SAM) to their histone substrates [6] . Lysine methylation occurs in three different product variations, mono-, di and trimethylation (me1, me2 and me3), which can have distinct biological functions [7] , [8] , [9] . Lysine methyltransferases (KMTs) are generally classified by the presence of a conserved SET (Su(var)3–9, Enhancer-of-zeste and Trithorax) domain [10] , [11] with the exception of enzymes of the DOT1 (disruption of telomeric silencing 1) family [12] , [13] . DOT1 was initially discovered in Saccharomyces cerevisiae [14] and subsequent sequence analysis revealed SAM-binding motifs that are characteristic for KMTs [15] . Transfer of the SAM methyl group to the ε-amino group of histone H3K79 is exclusively mediated by DOT1 enzymes [16] , [17] , [18] , [19] . Notably, H3K79 is located within the histone fold domain, explaining why DOT1 enzymes are strictly dependent on a nucleosomal context and cannot methylate free histone H3 proteins [16] , [17] , [18] , [19] . Crystal structures of the catalytic domain of yeast and human DOT1 enzymes revealed details of the interaction with the cofactor SAM and allowed the prediction of the location of a putative substrate-binding channel [20] , [21] . However, due to the challenging task to reconstitute a DOT1/nucleosome complex for structural studies, knowledge of the molecular basis for product specificity of these enzymes is currently very limited. In contrast, combinations of structure studies and mutational analysis of SET KMTs have been very successful in determining the molecular mechanism of their catalytic activity [22] , [23] , [24] , [25] , [26] , [27] , [28] . We used Trypanosoma brucei , a unicellular parasitic eukaryote that causes African sleeping sickness, as a model system to shed light on the methylation state-specific action of DOT1 enzymes. Interestingly, unlike most other eukaryotes, which possess only a single DOT1 enzyme, trypanosomes have two homologues, DOT1A and DOT1B, which methylate histone H3 on lysine 76, the homologous residue to H3K79 in other organisms. Notably, DOT1A and DOT1B have been shown to differ in their product specificity. Although DOT1A mediates mono- and dimethylation of H3K76, only DOT1B is able to catalyse H3K76 trimethylation [29] . Different methylation levels exhibit completely different functions in trypanosomes. DOT1A-mediated H3K76me1/me2 seems to regulate replication initiation [30] , which has also been shown for higher eukaryotes recently [31] , [32] . In contrast, H3K76me3 appears to be involved in transcriptional regulation [33] and developmental differentiation [29] . Similar functions were also suggested for DOT1 enzymes during development of higher eukaryotes [34] . In most cases, however, it is unclear whether the mono-, di- or trimethylated state is needed for the proper execution of these biological processes, because only one enzyme is responsible for all different methylation states. Hence, T. brucei is an extremely useful model organism to unravel the function and regulation of individual histone lysine methylation states. With this study we aim to understand the molecular basis of generating different methylation patterns on H3K76. We developed an in vitro trypanosomal reconstituted nucleosome system to investigate DOT1A and DOT1B methyltransferase activities under defined in vitro conditions. We exploit the unique feature of two different product specificities of the trypanosome DOT1 proteins to gain insights into the molecular mechanism of these important enzymes. Homology modelling allows us to identify amino acids (aa) within and outside of the catalytic centre that determine product specificity or influence catalysis rates. Functional mutational studies confirm the novel insights from our structural analysis, because exchange of critical aa transfers the product specificity of DOT1B to DOT1A. Moreover, despite the high degree of conservation of DOT1 methyltransferases among different eukaryotes, regulation of product specificity by regions distant from the catalytic site appears to be specific for trypanosomal DOT1 proteins. Our results have far-reaching implications for structural and functional studies of DOT1 enzymes in trypanosomes but also in other eukaryotes. Characterization of DOT1 using reconstituted nucleosomes The DOT1 target lysine K76 is located within the L1 loop connecting helices α1 and α2 of the conserved H3 histone fold ( Supplementary Fig. 1a ). Methylation of K76 by DOT1 does not work on purified histone H3 or short H3 peptides [16] , [21] , [29] , [35] , but rather depends on a structurally intact nucleosomal core surface [16] , [17] , [29] , [36] . Until now, in vitro studies of trypanosomal DOT1 enzymes were limited by the absence of a defined substrate. Attempts to reconstitute nucleosomes from trypanosomes remained unsuccessful so far and the essential character of DOT1A prevented purification of nucleosomes with unmodified H3K76 directly from the parasite cell [29] . Previous studies of trypanosomal DOT1 proteins relied on yeast nucleosomes as a substrate in a heterologous expression system, which could initially reveal different enzymatic activities but did not reflect exactly the situation in trypanosomes [37] . Although histones are in general highly conserved among different eukaryote species, the L1 loop of H3 containing the DOT1 target lysine K76 differs significantly in T. brucei [29] , [37] ( Supplementary Fig. 1a ). A closer examination revealed that differences extend beyond the H3 L1 loop and affect all four histones ( Supplementary Fig. 1 ), resulting in a markedly different nucleosome surface in T. brucei ( Supplementary Fig. 2 ). Moreover, it has been suggested that the human DOT1L enzyme binds to the nucleosome via interactions with all four core histones [20] , underlining the importance of a proper substrate for thorough enzymatic analysis of T. brucei DOT1 proteins. To circumvent the problems associated with artificial substrates, we established an in vitro nucleosome reconstitution system to characterize the intrinsic activity of both DOT1 enzymes. Full-length core histones (H2A, H2B, H3 and H4) from T. brucei were individually expressed in Echerichia coli , purified and refolded into octameric complexes, containing two copies of each histone ( Fig. 1a ). To generate mononucleosomes, octamers were assembled together with a specific 200 bp DNA fragment (601 sequence) optimized to bind histone octamers at a defined position [38] ( Fig. 1b ). Next, we used purified recombinant DOT1A and DOT1B wild-type (WT) proteins to test their intrinsic activity on the nucleosomal substrate. As controls, we mutated the central glycine residue of the DxGxGxG signature motif to arginine (G138R and G121R for DOT1A and DOT1B, respectively), generating catalytically inactive enzymes [29] , [37] . A histone methyltransferase assay was performed and H3K76 methylation levels (me1, me2 and me3) were detected by western blot analysis using specific antibodies [29] , [30] . Consistent with our previous observations [30] , DOT1A WT, but not its catalytically inactive G138R mutant, mono- and dimethylates H3K76 ( Fig. 1c ). In contrast, the DOT1B WT enzyme is able to catalyse all three methylation states on H3K76 ( Fig. 1c ), thereby extending its known repertoire by mono- and dimethylation on its natural substrate. In summary, we have successfully established an in vitro trypanosomal nucleosome-based methylation assay to investigate the distinct product specificity of DOT1. 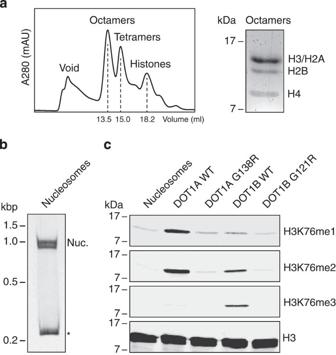Figure 1: Trypanosomal nucleosome reconstitution system reveals the intrinsic catalytic activity of DOT1A and DOT1B. (a) Octamers were refolded from purified recombinant histones and subjected to size-exclusion chromatography to separate tetramers and free histones (left panel). Pooled octamer fractions were analysed by SDS–PAGE (right) (H3 (14.8 kDa), H2A (14.2 kDa), H2B (12.6 kDa) and H4 (11.1 kDa). (b) Nucleosome assembly was analysed by gel mobility-shift assay on a native polyacrylamide gel. Nucleosomes (Nuc.) are separated from free DNA (marked with asterisk). (c) Enzymatic activity of purifiedT. bruceiwild-type DOT1A and DOT1B, and catalytically inactive mutants (DOT1A G138R and DOT1B G121R) was tested on reconstituted nucleosomesin vitro. After western blotting, different methylation states were detected with specific antibodies. H3 signals serve as loading control. Figure 1: Trypanosomal nucleosome reconstitution system reveals the intrinsic catalytic activity of DOT1A and DOT1B. ( a ) Octamers were refolded from purified recombinant histones and subjected to size-exclusion chromatography to separate tetramers and free histones (left panel). Pooled octamer fractions were analysed by SDS–PAGE (right) (H3 (14.8 kDa), H2A (14.2 kDa), H2B (12.6 kDa) and H4 (11.1 kDa). ( b ) Nucleosome assembly was analysed by gel mobility-shift assay on a native polyacrylamide gel. Nucleosomes (Nuc.) are separated from free DNA (marked with asterisk). ( c ) Enzymatic activity of purified T. brucei wild-type DOT1A and DOT1B, and catalytically inactive mutants (DOT1A G138R and DOT1B G121R) was tested on reconstituted nucleosomes in vitro . After western blotting, different methylation states were detected with specific antibodies. H3 signals serve as loading control. Full size image DOT1A and DOT1B are distributive enzymes in vitro KMTs can either work in a processive or distributive manner. Processive enzymes set multiple modifications on the substrate lysine without dissociation, and therefore intermediate methylation states might not be observed. In contrast, distributive enzymes are only able to transfer one methyl group to the substrate per binding event, resulting in detectable intermediates. Indeed, a complex methylation pattern in vivo with simultaneous presence of me1, me2 and me3 states has been interpreted as being indicative for a distributive enzyme [39] . Notably, yeast and human DOT1 crystal structures show separate lysine- and SAM-binding channels, consistent with the possibility of a processive catalytic mode of action because the cofactor SAM can be exchanged without dissociation from the substrate [20] , [21] . To determine the catalytic mode, we performed methyltransferase assays with both trypanosomal DOT1 proteins using increasing enzyme concentrations for a fixed period of time as previously described for yeast Dot1p [39] . With a constant assay time, the two possible methylation patterns are characteristic for the enzyme’s mode of action. Increasing amounts of a processive enzyme produce increasing amounts of methylated H3K76, but the relative abundance of the different methylation states should be invariant. In contrast, a distributive enzyme is expected to first monomethylate several lysines before it re-associates with monomethylated lysines to introduce a second methyl group. Similarly, an accumulation of H3K76 dimethylation should be observed before trimethylated lysine is detectable. Therefore, the relative abundance of the three different methylation states should change with increasing amount of distributive enzyme. In our assay, low concentrations of DOT1A lead to a weak H3K76 monomethylation signal, whereas increased amounts result in the accumulation of me1, which is a prerequisite for the transition to me2 ( Fig. 2a ). The independent me1 and me2 product waves, hence, the different ratios of methylations states, are characteristic for a distributive enzyme. Similar results were obtained for DOT1B, where me1, me2 and me3 products follow each other in consecutive waves with increasing enzyme concentrations ( Fig. 2b ). Based on these results, we conclude that both trypanosomal DOT1 KMTs use a distributive mechanism to methylate H3K76 in vitro . 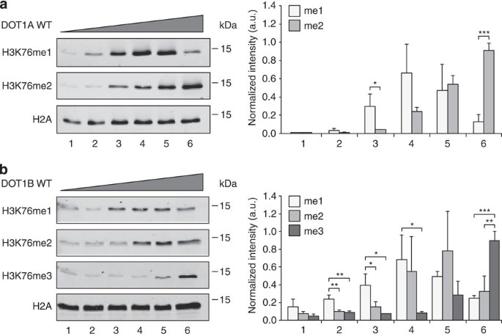Figure 2: DOT1A and DOT1B are distributive enzymesin vitro. Histone methyltransferase assays were carried out for DOT1A (a) and DOT1B (b) with increasing enzyme concentrations (0.1–100 ng μl−1, samples 1–6) and a fixed time of 2 h. Methylation states were analysed by western blotting (left) and quantified to allow statistical evaluation (right). Data are shown as means±s.d. (n=3). Statistical significance is indicated (*P<0.05, **P<0.01, ***P<0.001, two-tailed Student’st-test). Figure 2: DOT1A and DOT1B are distributive enzymes in vitro . Histone methyltransferase assays were carried out for DOT1A ( a ) and DOT1B ( b ) with increasing enzyme concentrations (0.1–100 ng μl −1 , samples 1–6) and a fixed time of 2 h. Methylation states were analysed by western blotting (left) and quantified to allow statistical evaluation (right). Data are shown as means±s.d. ( n =3). Statistical significance is indicated (* P <0.05, ** P <0.01, *** P <0.001, two-tailed Student’s t -test). Full size image DOT1 structure homology modelling Next, we wanted to understand the molecular basis for the different product specificities of DOT1A and DOT1B observed in vivo and in vitro [29] , [30] ( Fig. 1c ). DOT1 enzymes differ dramatically in size in different eukaryotes, ranging from 582 aa in yeast, over 1537 aa in humans to 2137 aa in the fruit fly ( Supplementary Fig. 3a ). Length variations result mainly from species-specific amino- and carboxy-terminal extensions outside the conserved KMTase domain, parts of which are required for effective nucleosome interaction by providing a DNA binding interface [20] , [21] . T. brucei DOT1A (295 aa) and DOT1B (275 aa) appear to lack these extensions and comprise only the KMTase catalytic core ( Supplementary Fig. 3a ). Compared with the human DOT1L enzyme, the catalytic cores of DOT1A and DOT1B share 20% and 22% sequence identity, and 33% and 32% similarity, respectively ( Fig. 3a ). Based on the high degree of conservation, we generated homology models of the T. brucei proteins using the human DOT1L crystal structure as template [20] . The models include residues 79–295 and 62–275 for DOT1A and DOT1B, respectively ( Fig. 3a,b and Supplementary Fig. 3b,c ) and cover the C-terminal open α/β domain, formed by seven β-strands (β5–β11) that are flanked by five α-helices (αF–αJ) ( Supplementary Data 1 and 2 ). This C-terminal part of the KMTase domain is linked to N-terminal helices (αD and αE) via the loop EF ( Fig. 3a,b and Supplementary Fig. 3b,c ). DOT1A and DOT1B have an acidic patch close to the active site ( Supplementary Fig. 4a ), which is absent in DOT1 enzymes of other organisms. The patch is formed by D247/D248 and E226/D227 residues in DOT1A and DOT1B, respectively, and is conserved among trypanosomal DOT1 enzymes ( Supplementary Fig. 5 ). We suggest that this negatively charged patch might be the binding counterpart of the positively charged residues around H3K76 ( Supplementary Fig. 4b ) and contributes to nucleosome targeting. Non-SET domain methyltransferases such as DOT1 are characterized by a series of conserved motifs (I, I’ and II) [15] , [40] and the corresponding regions are also present in T. brucei DOT1A and DOT1B ( Fig. 3a and Supplementary Table 1 ). Two motifs, D1 and D2, appear to be specific for the DOT1 family of methyltransferases [20] . Although the D2 motif is present but less conserved in T. brucei DOT1A and DOT1B, it has been proposed that the D1 motif is absent from trypanosomal DOT1 enzymes [29] . Residues from all motifs (I, I’, II, D1 and D2) are involved in co-factor binding and/or in formation of the target lysine-binding channel of DOT1 proteins [20] , [21] ( Fig. 3a and Supplementary Table 1 ). The D1 motif forms a significant part of the substrate-binding pocket [20] , [21] and we wondered which part of the trypanosomal DOT1 enzymes could take over this function. Alignments allowed us to identify a sequence (CAKS, single letter aa code) that is nearly invariant across trypanosomes, suggesting conserved functional importance ( Supplementary Fig. 5 ). We aligned the CAKS sequence in our homology models under the D1 motif of other eukaryotes (YGET sequence) ( Fig. 3a ) based on the following structural arguments: (i) the small alanine side chain (A109 (DOT1A), A92 (DOT1B)) is positioned where other eukaryotic DOT1 enzymes have a glycine residue that has been proposed to be critical to maintain an open lysine-binding channel [20] , [21] ( Fig. 3a and Supplementary Table 1 ); (ii) placement of the lysine residue (K110 (DOT1A), K93 (DOT1B)) positions the positively charged side chain away from the substrate-binding channel that otherwise might cause electrostatic repulsion of the target lysine ( Fig. 3c ); and (iii) the serine side chain (S111 (DOT1A) and S94 (DOT1B)) can stabilize the SAM carboxyl group via a hydrogen bond according to the function of threonine at this position in human DOT1L [20] ( Fig. 3a and Supplementary Table 1 ). Taken together, we present a structure-guided DOT1 sequence alignment based on homology modelling ( Fig. 3a ), which includes significant improvements compared with a previous effort [29] and propose that the CAKS sequence forms the trypanosomal D1 motif that generates part of the substrate-binding channel ( Fig. 3c ). 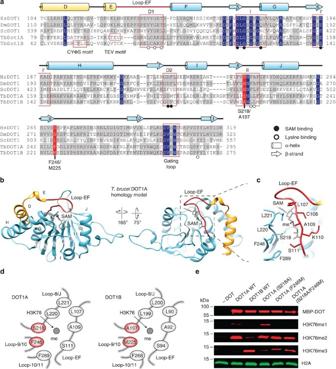Figure 3: Structure-guided mutations identify residues sufficient for product specificity of DOT1A and DOT1B. (a) Improved structure-guided sequence alignment of the conserved DOT1 methyltransferase domain from Hs (H. sapiens, gene identifier (GI): 22094135)20, Dm (Drosophila melanogaster, GI: 320542472), Sc (S. cerevisiae, GI: 6320648)21and Tb (T. brucei, GI: 72392449 (DOT1A), GI: 115503935 (DOT1B)). Invariant aa positions are highlighted (white letter against dark blue background), conserved residues are indicated with grey background. Secondary structure elements (α-helices D to J and β-strands 5 to 11) of the human enzyme are shown20. Conserved DOT1 motifs (I, I’, II, D1, D2 and gating loop) are indicated. Open and closed circles mark residues implicated in lysine and SAM binding, respectively. Positions of mutants (S218, F246 (DOT1A) and A197, M225 (DOT1B)) are highlighted in red. (b) Homology model of the DOT1A catalytic core domain viewed from the entrances of the SAM- (left panel) and lysine- (right panel) binding pockets. Model is coloured as ina. (c) Close-up view of the lysine-binding pocket of DOT1A. (d) Schematic representation of the aa forming the H3K76-binding channel inT. bruceiDOT1A (left) and DOT1B (right) leading to the methyl group (me) of SAM. Residues that differ between the two enzymes are highlighted in red. (e) Enzymatic activity of purifiedT. bruceiDOT1A mutants (S218A, F246M and S218A/F246M) were tested on reconstituted nucleosomesin vitro. H2A signals serve as loading control. Figure 3: Structure-guided mutations identify residues sufficient for product specificity of DOT1A and DOT1B. ( a ) Improved structure-guided sequence alignment of the conserved DOT1 methyltransferase domain from Hs ( H. sapiens , gene identifier (GI): 22094135) [20] , Dm ( Drosophila melanogaster , GI: 320542472), Sc ( S. cerevisiae , GI: 6320648) [21] and Tb ( T. brucei , GI: 72392449 (DOT1A), GI: 115503935 (DOT1B)). Invariant aa positions are highlighted (white letter against dark blue background), conserved residues are indicated with grey background. Secondary structure elements (α-helices D to J and β-strands 5 to 11) of the human enzyme are shown [20] . Conserved DOT1 motifs (I, I’, II, D1, D2 and gating loop) are indicated. Open and closed circles mark residues implicated in lysine and SAM binding, respectively. Positions of mutants (S218, F246 (DOT1A) and A197, M225 (DOT1B)) are highlighted in red. ( b ) Homology model of the DOT1A catalytic core domain viewed from the entrances of the SAM- (left panel) and lysine- (right panel) binding pockets. Model is coloured as in a . ( c ) Close-up view of the lysine-binding pocket of DOT1A. ( d ) Schematic representation of the aa forming the H3K76-binding channel in T. brucei DOT1A (left) and DOT1B (right) leading to the methyl group (me) of SAM. Residues that differ between the two enzymes are highlighted in red. ( e ) Enzymatic activity of purified T. brucei DOT1A mutants (S218A, F246M and S218A/F246M) were tested on reconstituted nucleosomes in vitro . H2A signals serve as loading control. Full size image Mutations change the product specificity of DOT1A A systematic comparison including the available yeast and human DOT1 crystal structures [20] , [21] allowed us to identify eight residues that form a putative substrate-binding channel in T. brucei DOT1A (S111, S218, F246, F289, L107, A109, L220 and L221) and DOT1B (S94, A197, M225, F268, L90, A92, L199 and L200), which directly leads to the SAM methyl group as it has been proposed for yeast and human DOT1 proteins [20] , [21] ( Fig. 3c,d and Supplementary Table 1 ). Among these eight aa, two differ between both enzymes and are located between loop 8/9 (S218 (DOT1A), A197 (DOT1B)) and loop 9/10 (F246 (DOT1A), M225 (DOT1B)) ( Fig. 3d and Supplementary Table 1 ). We decided to exchange these two positions in DOT1A with the corresponding residues of DOT1B to test our hypothesis that these aa are responsible for the distinguishable product specificity. The resulting mutant enzymes (DOT1A S218A and F246M) were purified and tested in our in vitro methyltransferase assay. The results clearly demonstrate that both single mutations are sufficient to confer DOT1B-specific trimethylation activity to DOT1A ( Fig. 3e ). Combination of both exchanges in a double mutant (DOT1A S218A/F246M) further increased the me3 signal to almost DOT1B WT level ( Fig. 3e ). We noticed that the DOT1A F246M mutant showed no me1 signal in comparison with DOT1A WT and the S218A mutant enzyme, indicating that the F246M mutation might affect the reaction rate of H3K76 dimethylation ( Fig. 3e ). To further explore this observation, we monitored me1 and me2 accumulation for DOT1A WT and the F246M mutant over time ( Supplementary Fig. 6 ). Interestingly, although the conversion of me0 to me1 showed no differences, the subsequent reaction to produce me2 appears to proceed significantly faster in the presence of the DOT1A F246M mutant ( Supplementary Fig. 6 ). Taken together, these results provide experimental support for the proposed structure of the substrate-lysine channel [20] , [21] . Furthermore, they establish a novel function for two aa positions in DOT1 enzymes in determining the distinct methylation product specificity and/or reaction rate. The N-terminal region affects the lysine-binding channel As the H3K76me3 signal generated by the DOT1A S218A/F246M double mutant did not reach DOT1B WT level ( Fig. 3e ), we wondered what additional components outside of the lysine-binding channel could influence the catalytic activity of the enzyme. Yeast and human DOT1 crystal structures revealed that the N- and C-terminal parts of the KMTase domain are in close vicinity to each other, and that the interface appears to stabilize the lysine-binding pocket [20] , [21] . Notably, the corresponding N-terminal parts of T. brucei DOT1A and DOT1B differ significantly between each other ( Figs 3a and 4a ), possibly affecting the substrate-binding site geometries that contribute to the distinct product specificities. We decided to exchange the N-terminal part of DOT1A (residues 1–102) with the corresponding sequence from DOT1B (residues 1–85) in WT and S218A/F246M mutant background. The chimeric WT enzyme produced only monomethylated H3K76 and all chimeric mutants were catalytically inactive ( Fig. 4b ). Importantly, the enzyme chimeras are very likely to be properly folded, as me1 activity is maintained in the chimeric DOT1A WT protein ( Fig. 4b ). These results indicate a contribution of the DOT1 N terminus to the formation of the catalytic active site of the enzyme. However, exchanging the entire N-terminal region probably affects a wide range of contacts with the conserved C-terminal part (for example, interactions of helices αD and αH ( Fig. 3b and Supplementary Fig. 3b )) and thus could explain the catalytically inactive mutant DOT1A chimeras ( Fig. 4b ). This suggests that the N-terminal part contributes to lysine-binding channel formation via a small set of residues at the interface between the N- and C-terminal parts of the KMTase domain. Sequence alignment of several putative DOT1A and DOT1B sequences from various trypanosome species revealed two conserved residue stretches located N-terminally of the D1 motif. These motifs appear to be specific for either DOT1A (TEV sequence) or DOT1B (CYΦS sequence, where Φ represents hydrophobic aa) ( Fig. 4a , Supplementary Fig. 5 and Supplementary Table 2 ). Interestingly, our homology models allowed the prediction that both of these stretches are pointing towards the common D1 motif (CAKS sequence) within loop EF, which forms one side of the target lysine-binding channel ( Figs 3c and 4a ). The equivalent tyrosine of the CYΦS motif is conserved in yeast, fly and human DOT1 enzymes ( Fig. 3a and Supplementary Table 2 ), where it participates in a hydrogen bond network to stabilize the D1 motif [20] , [21] . We speculated that the trypanosomal N-terminal sequence motifs are used to alter the lysine-binding channel geometry via different hydrogen bond interactions with the common central lysine residue (K110 in DOT1A and K93 in DOT1B) of the trypanosome D1 motif ( Fig. 4a ). To test our hypothesis, we exchanged the possible hydrogen-bonding positions in DOT1A (F90/E100) with the corresponding residues of DOT1B (Y73/T83) in WT and S218A/F246M mutant background (DOT1A (FE) and DOT1A (SF-FE) mutants, respectively). Swapping the putative hydrogen-bonding residues conferred trimethylation activity to DOT1A, revealing a significant influence of distant parts on the catalytic centre of the enzyme ( Fig. 4c ). Notably, the F90Y mutation introduces a tyrosine at the exact same position, where yeast and human DOT1 proteins contain their hydrogen-bonding tyrosine, indicating that this conserved residue is a universal hallmark of trimethylating DOT1 enzymes. Furthermore, we introduced the majority of the DOT1B CYΦS motif in DOT1A, while simultaneously removing the TEV motif (T89C, F90Y, R92S, T99V and E100T) in the WT and S218A/F246M mutant background (DOT1A (TFRTE) and DOT1A (SF-TFRTE) mutants) to clarify whether residues beyond the possible hydrogen-bonding positions also have an influence on the efficiency of trimethylation. However, no apparent increase in trimethylation signals can be observed for these multiple mutants ( Fig. 4c ). Taken together, our results allowed us to define two sequence motifs (TEV and CYΦS) within the N-terminal region of the KMTase domain that are specific for either DOT1A or DOT1B enzymes and are crucial in determining their distinct product specificities. 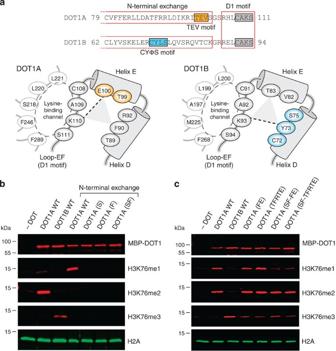Figure 4: The N-terminal part of the DOT1 KMTase domain contributes to formation of the lysine-binding pocket. (a) The aa sequence (upper panel) and schematic representation of the N-terminal regions with signature motifs (lower panel) of DOT1A and DOT1B enzymes. Highlighted are CAKS (grey), TEV (orange) and CYΦS (blue). Range of the D1 motif and N-terminal exchange are marked with red boxes. The proposed differences in stabilization of the lysine-binding pocket by hydrogen bonds in DOT1A and DOT1B are indicated with dashed lines. (b) Enzymatic activity of purified DOT1A mutants (S218A, F246M and S218A/F246M) with residues 1–102 exchanged with the corresponding sequence from DOT1B (residues 1–85) was tested on reconstituted nucleosomes. H2A signals serve as loading control. (c) Activity of DOT1A double and quintuple mutants (DOT1A E100T/F90Y (DOT1A FE) and DOT1A T89C/F90Y/R92S/T99V/E100T (DOT1A TFRTE), respectively), in WT and S218A/F246M mutant background, were tested on reconstituted nucleosomes. H2A signals serve as loading control. Figure 4: The N-terminal part of the DOT1 KMTase domain contributes to formation of the lysine-binding pocket. ( a ) The aa sequence (upper panel) and schematic representation of the N-terminal regions with signature motifs (lower panel) of DOT1A and DOT1B enzymes. Highlighted are CAKS (grey), TEV (orange) and CYΦS (blue). Range of the D1 motif and N-terminal exchange are marked with red boxes. The proposed differences in stabilization of the lysine-binding pocket by hydrogen bonds in DOT1A and DOT1B are indicated with dashed lines. ( b ) Enzymatic activity of purified DOT1A mutants (S218A, F246M and S218A/F246M) with residues 1–102 exchanged with the corresponding sequence from DOT1B (residues 1–85) was tested on reconstituted nucleosomes. H2A signals serve as loading control. ( c ) Activity of DOT1A double and quintuple mutants (DOT1A E100T/F90Y (DOT1A FE) and DOT1A T89C/F90Y/R92S/T99V/E100T (DOT1A TFRTE), respectively), in WT and S218A/F246M mutant background, were tested on reconstituted nucleosomes. H2A signals serve as loading control. Full size image An important factor for the DOT1 catalytic mechanism is deprotonation of the target lysine ε-amine to produce a lone electron pair that can initiate the nucleophilic attack on the methylsulfonyl group of SAM. The resulting methyl lysine further undergoes consecutive rounds of methylation, which requires repeated deprotonation in combination with a rotation of the target lysine side chain. Differences in the local environment of DOT1A and DOT1B that influence deprotonation could in principle account for the varying product specificities. One factor favouring deprotonation is an overall hydrophobic environment [41] in combination with negative charges in the proximity of the target lysine that could take up the proton. Although the molecular details remain to be determined, both T. brucei DOT1 enzymes are likely to behave similar to human and yeast DOT1s with respect to the deprotonation step. The lysine-binding channel has a hydrophobic entrance and an overall negative charge at the base in all DOT1 enzymes analysed to date. No specific negatively charged residue is present in the channel, but the overall negative charge has been proposed to achieve deprotonation [20] , [21] analogous to the situation in SET domain-containing methyltransferases [23] . In addition, the SAM carboxylate group may contribute to deprotonation of the target lysine, as it is not compensated by a positive charge in its immediate proximity. Taken together, we propose that differences in the lysine deprotonation step are very unlikely to exist for DOT1A and DOT1B, and product specificity is determined by other means. First insights into the structural determinants of product specificity came from comparisons of the SET domain containing KMTs DIM-5 and SET7/9, which catalyse formation of distinct products (me1/2/3 for DIM-5 and me1 for SET7/9) [42] . A single position occupied by either a phenylalanine (in DIM-5) or a tyrosine (in SET7/9) determines product specificity in these cases and swapping the residues changes product specificity of the mutant enzymes [42] . We hypothesize that S218 in DOT1A functions in a related fashion by hydrogen bonding to the target lysine ε-amine and thus restricting the enzyme activity to mono- and dimethylation of H3K76. The S218A mutation removes the hydroxyl group, which would allow free rotation of the target lysine and consequently the mutant enzyme is able to set the trimethylation mark. This scenario resembles the situation in the SET7/9 methyltransferase, where hydrogen bonding of two tyrosines restricts rotation of the substrate lysine and thus limits the product to me1 (ref. 26 ). F246 of T. brucei DOT1A might restrict the target lysine movement or cause steric exclusion of a trimethylated lysine via its bulky aromatic side chain. The F246M mutation introduces a smaller side chain and confers more space for the substrate lysine, which might be a prerequisite for the trimethylation activity of DOT1B. Notably, an F379M mutation in the active site of the arginine methyltransferase PRMT5 from Caenorhabditis elegans resulted in a relaxed product specificity [43] , resembling the situation in T. brucei DOT1A. However, superimposition of the PRMT5 crystal structure [43] with our DOT1A homology model revealed that the two phenylalanine residues are approaching the cofactor SAM from opposite sides. This indicates that the altered product specificities provided by the phenylalanine to methionine mutations are a consequence of more conformational flexibility and relaxed steric constraints within the active sites and not due to the precise positioning of the phenylalanine residues with respect to SAM. The T. brucei DOT1A F246M mutation not only changes the product specificity but also increases the reaction rate of di- but not monomethylation, indicating that a monomethylated lysine is a better substrate for the DOT1A F246M mutant compared with the WT enzyme. DOT1A F246 is located in close proximity to F116 and F289 on one side of the lysine-binding channel. Notably, recognition and binding of methylated lysines often involve so-called aromatic cages found in members of the Royal superfamily of folds (for example, chromo- and tudor domains) and plant homeo domain (PHD) fingers [44] . DOT1A F246 together with F116 and/or F289 might form an aromatic cage-like structure that could function as a temporal trap for H3K76me1. Such a trap close to the active site could effectively slow down the dimethylation reaction, without affecting monomethylation. In contrast, the F246 equivalent M225 in DOT1B cannot form an aromatic cage, which is consistent with our results showing that DOT1B is more effective in converting lower to higher methylation states compared with DOT1A ( Fig. 3c ). This observation is perfectly compatible with the different functions of DOT1A and DOT1B in the parasite. DOT1A-mediated H3K76me1/2 appears slowly after incorporation of new H3 into the chromatin fibre restricting these marks to G2 phase and mitosis, whereas DOT1B seems to convert all H3K76 quickly to a trimethylated state at the end of mitosis [30] . The importance of lysine-binding pocket stabilization by N-terminal parts of the KMTase domain has been previously established by structural work on yeast and human DOT1 enzymes [20] , [21] . Here, the central glutamate (E374 in S. cerevisiae and E138 in Homo sapiens ) of the D1 motif is engaged in a hydrogen bond with an N-terminal tyrosine (Y350 and Y115 in S. cerevisiae and H. sapiens , respectively). Disrupting or changing the hydrogen-bonding properties at this position by E374Q or E374A mutations abolishes enzymatic activity of the yeast Dot1 enzyme [21] . Moreover, a Y350F mutation in yeast dramatically reduces DOT1 activity, underlining the importance of the tyrosine hydroxyl group for positioning E374 via a hydrogen bond, thus maintaining a proper architecture of the lysine-binding pocket [21] . Our results clearly establish a novel function for the N-terminal part of the KMTase core in determining product specificity of DOT1 enzymes by variation of the interaction pattern with the conserved D1 motif. This offers the interesting possibility to alter the D1 stabilization via the N-terminal region in organisms containing a single DOT1 enzyme to specifically change product specificity. For example, a DOT1 mutant that only mediates mono- or dimethylation of H3K79 in yeast could be an extremely useful tool to address the still discussed possibility of functional redundancy of different methylation levels. In conclusion, we successfully exploited the different enzymatic activities of trypanosome DOT1 homologues to identify several structural components that are responsible for product specificity of these conserved histone methyltransferases. This does not only shed light on the mode of action of the parasites enzymes but might also help to understand the function and regulation of members of the DOT1 family in other eukaryotes. This information could be useful to generate DOT1 mutants with specific enzymatic activities to solve long-standing questions about possible redundancy of different methylation states. Purification of DOT1 T. brucei DOT1A (TriTryp database ID: Tb927.8.1920) and DOT1B (Tb927.1.570) coding sequences were amplified by PCR from genomic DNA using following primers: DOT1A_for 5′-ATGCCTGGATTGCTAATATCCCGG-3′, DOT1A_rev 5′-CCCCAAGCTTTCATCTCCGTCGGTGAATGAAAAAAGG-3′, DOT1B_for 5′-ATGGACGCACGTGTTCATCGTAGTAAGC-3′ and DOT1B_rev 5′-CCCCAAGCTTTCACGATCGCTTGATGTAAAGATAAAATGG-3′. Full-length DOT1A and DOT1B open reading frames were cloned into the pMAL-c2X expression vector (New England Biolabs) using Hind III and Xmn I restriction sites, resulting in N-terminal fusions to the maltose-binding protein (MBP). Mutations were introduced using site-directed mutagenesis following standard procedures. Vectors were transformed into E. coli Rosetta Blue (Novagen) and cells were grown in selective media (Luria–Bertani medium supplemented with 100 μg ml −1 ampicillin and 34 μg ml −1 chloramphenicol) to an OD 600 of 0.5–0.6 before induction of protein expression with 1 mM isopropyl-β- D -thiogalacto-pyranoside for 2.5 h at 28 °C. Cells were harvested (8,000 g , 15 min, 4 °C) and lysed in buffer A (20 mM Tris-HCl pH 7.4, 200 mM NaCl, 1 mM Na-EDTA) using a Bioruptor (Diagenode). MBP fusion proteins were purified from the cleared lysate by affinity chromatography using amylose resin (New England Biolabs) and eluted with 1 mM maltose after extensive washing with Buffer A. Purification of histone proteins T. brucei full-length histone open reading frames of H2A (TriTryp database ID: Tb927.7.2850), H2B (Tb927.10.10510), H3 (Tb927.1.2510) and H4 (Tb927.5.4170) were amplified by PCR from genomic DNA using following primers: H2A_for 5′-AGATCATATGGCAACACCCAAACAGGC-3′, H2A_rev 5′-ATCTCGAGCTAGACGCTTGGCGTCGCC-3′, H2B_for 5′-AGATCATATGGCCACTCCTAAGAGCAC-3′, H2B_rev 5′-ATCTCGAGCTAGCTGGAAGCGTGTGACAC-3′, H3_for 5′-AGATCATATGTCGAGGACCAAGGAAAC-3′, H3_rev 5′-ATCTCGAGCTATGCACGTTCACCGCGTAG-3′, H4_for 5′-CGCCATATGGCGAAGGGTAAGAAGAGTGGT-3′, H4_rev 5′-CGGAATTCCTATGCATAACCGTACAGAATCTT-3′. PCR products were cloned into the pET21a(+) vector (Novagen) using Nde I and Xho I restriction sites for H2A, H2B and H3, and Nde I and EcoR I for H4. All vectors were individually transformed into Rosetta BL21 (DE3) E. coli strain and cells were grown in selective media (Luria–Bertani medium supplemented with 100 μg ml −1 ampicillin, 1% (v/v) glucose) to an OD 600 of 0.6 before induction of protein expression with 1 mM isopropyl-β- D -thiogalacto-pyranoside for 3 h at 37 °C. Histones were purified from inclusion bodies essentially following the protocol from Luger et al. [45] Briefly, cells were harvested (8000 g , 15 min, 4 °C) and lysed in histone wash buffer (HWB) (50 mM Tris-HCl pH 7.5, 100 mM NaCl, 1 mM EDTA, 1 mM benzamidine, 5 mM β-mercaptoethanol) by sonication using a Bioruptor (Diagenode) with high-power settings in 30 s on/off cycles for 10 min. The inclusion body-containing cell fraction was harvested (23,000 g , 20 min, 4 °C), resuspended in HWB supplemented with 1% (v/v) Triton X-100 (HWB/T) and sonicated as described above. The purification steps (resuspension, sonification and harvest) were repeated once in HWB/T and twice in HWB. After the final purification step, inclusion bodies were resuspended in unfolding buffer (7 M guanidinium chloride, 20 mM Tris-HCl pH 7.5, 10 mM dithiothreitol (DTT)) for 1 h at 20 °C and separated from remaining cell debris by centrifugation (23,000 g , 15 min, 4 °C). Unfolded proteins were dialysed against SAU-200 buffer (7 M urea, 20 mM Na(OAc) pH 5.2, 200 mM NaCl, 1 mM EDTA, 5 mM β-mercaptoethanol). Proteins were separated from precipitates by centrifugation (23,000 g , 15 min, 4 °C) and applied on a HiTrap SP HP cation exchange column (GE Healthcare) in SAU-200 buffer. Histone proteins were eluted from the column using a salt gradient from 200 to 600 mM NaCl in SAU buffer (7 M urea, 20 mM Na(OAc) pH 5.2, 1 mM EDTA, 5 mM β-mercaptoethanol). Purified histones were dialysed against distilled water containing 2 mM β-mercaptoethanol and lyophilized using an Alpha 1–2 LD freeze dryer (Christ). Nucleosome assembly Nucleosomes were assembled with refolded histones in principle as described [46] . Core histone proteins were separately dissolved in unfolding buffer (7 M guanidinium chloride, 20 mM Tris-HCl pH 7.5, 10 mM DTT) to a final concentration of 2 mg ml −1 each and incubated for 30 min at 20 °C before mixing (H2A:H2B:H3:H4 in a molar ratio of 1.2:1.2:1:1). The total protein concentration of the sample was adjusted to 1 mg ml −1 with unfolding buffer, followed by dialysis against refolding buffer (10 mM Tris-HCl pH 7.5, 2 M NaCl, 1 mM EDTA, 5 mM β-mercaptoethanol) to allow histone octamer formation. The sample was concentrated using a Microcon-10 centrifugal filter unit (Millipore) before loading on a Superdex 75 10/300 size-exclusion chromatography column (GE Healthcare) in refolding buffer (10 mM Tris-HCl pH 7.5, 2 M NaCl, 1 mM EDTA, 5 mM β-mercaptoethanol). Histone octamer containing fractions were combined and concentrated to ~1 mg ml −1 using a Microcon-30 centrifugal filter unit (Millipore). In parallel, histone H2A/H2B dimers were separately collected during size-exclusion chromatography. Protein sample aliquots were frozen in liquid nitrogen and stored at −80 °C. All components required for nucleosome assembly (histone octamers, excess H2A/H2B dimers and 601 nucleosome positioning sequence [38] (kind gift from Daniela Rhodes)) were mixed in a 1:1.2:1 molar ratio in reconstitution buffer (20 mM Tris-HCl pH 7.5, 10 mM DTT, 1 mM EDTA, 2 M KCl, 0.5 mM benzamidine) and incubated on ice for 30 min. The samples were subsequently placed into dialysis tubing and transferred into high salt buffer (10 mM Tris-HCl pH 7.5, 2 M KCl, 1 mM EDTA, 1 mM DTT, 0.5 mM benzamidine), which was gradually replaced with low-salt buffer (10 mM Tris-HCl pH 7.5, 250 mM KCl, 1 mM EDTA, 1 mM DTT, 0.5 mM benzamidine) during a time window of 50 h at 4 °C using a peristaltic pump. Nucleosome samples were subsequently dialysed against TCS buffer (20 mM Tris/HCl pH 7.5, 1 mM EDTA, 1 mM DTT) supplemented with 15% (v/v) glycerol and stored at −80 °C. Methyltransferase assay Unless stated otherwise, 22.5 ng μl −1 nucleosomes were incubated with 30 ng μl −1 of purified DOT1A or DOT1B enzymes in reaction buffer (50 mM Tris-HCl pH 8.0, 50 mM KCl, 5 mM CaCl 2 , 100 mM NaCl, 2.5% (v/v) glycerol, 0.025% (v/v) NP-40, 0.5 mM DTT) in the presence of 2.5 mM SAM in an 80-μl assay. Samples were incubated for 1 or 3 h, or until completion of the reaction at 30 °C. Samples were analysed by SDS–PAGE and western blotting. Uncropped gels and blots are provided in Supplementary Figs 8–12 . Antibodies For western blot analysis, rabbit polyclonal peptide antibodies specific for mono-, di- or trimethylated trypanosomal histone H3K76 were used [29] , [30] (anti-TbH3K76me1: 1:1,000; anti-TbH3K76me2: 1:2,000; and anti-TbH3K76me3: 1:2,000, all from Sigma-Aldrich). Trypanosomal histones H2A and H3 were detected using polyclonal guinea pig (anti-TbH2A: 1:1,000, Pineda) and rabbit (anti-TbH3: 1:10,000, Pineda) [30] antibodies, respectively. Histone H2A and H3 antibodies were generated by immunization with full-length recombinant proteins. For detection of DOT1 enzymes via the MBP tag, a monoclonal rat antibody (anti-MBP IgG2a: 1:10,000, gift from E. Kremmer, Helmholtz Center Munich) [47] was used. Secondary antibody signals (goat anti-rabbit IRDye 800 CW: 1:50,000; donkey anti-guinea pig IRDye 800CW: 1:50,000; goat anti-rat IRDye 680LT: 1:50,000; and goat anti-rabbit 680LT: 1:50,000, all from LI-COR Biosciences) were detected with an Odyssey infrared imaging system (LI-COR Biosciences). Homology modelling Template searches were performed with HHpred [48] , which is based on the pairwise comparison of profile hidden Markov models [49] , using default settings and full-length T. brucei DOT1A and DOT1B sequences as input. Among the obtained results, the H. sapiens DOT1L crystal structure (protein data bank (PDB) accession number 1NW3) [20] was chosen as structural template for subsequent homology model building. The underlying alignments generated by HHpred had expected ( E )-values of 1.1e−25 and 6.9e−22 for DOT1A and DOT1B, respectively. Note that the S. cerevisiae Dot1p crystal structure (PDB accession number 1U2Z) [21] gave slightly better results in this search ( E -values of 5.7e−26 and 4.7e−23 for DOT1A and DOT1B, respectively). However, the yeast template was not chosen because of the loop β10–β11 interaction with the substrate-binding site observed in the Dot1p crystal structure [21] , which we assumed could pose unwanted restraints on the homology models. Similarity of the T. brucei DOT1 enzymes with the DOT1L sequence dropped considerably for the N-terminal parts of the enzymes prior residues 79 and 62 for DOT1A and DOT1B, respectively, which prevented extension of the homology models beyond this point. Repeated template searches with HHpred for the N-terminal residues only (1–78 and 1–61 for T. brucei DOT1A and DOT1B, respectively) did not provide statistical significant results (all obtained alignments had E -values much greater than 1). The conserved CAKS motif (residues 108–111 and 91–94 for T. brucei DOT1A and DOT1B, respectively) was manually re-aligned under the D1 motif of the human DOT1L enzyme according to the structural argumentation described in the main text. The DOT1 alignments obtained by HHpred were manually combined with the repositioned CAKS motif in Jalview [50] exported in the PIR alignment file format and manually fed in Modeller [51] with the human DOT1L crystal structure (PDB accession number 1NW3, residues 104–319) as template. The final T. brucei DOT1 homology models generated by Modeller covered residues 79–295 and 62–275 for DOT1A and DOT1B, respectively, and have root mean square deviations of 1.36 and 1.04 Å with respect to the human DOT1L crystal structure (on superposition of 212 α-carbons in both cases) with good geometries as indicated by a validation using PROCHECK [52] (91.3%/92.2% of DOT1A/DOT1B residues in most favoured, 8.2%/6.2% in additionally allowed, 0.5%/1.0% in generously allowed and 0.0%/0.5% in disallowed regions of the Ramachandran plot). Quality of the DOT1 homology models was further assessed with the QMEAN composite scoring function [53] , which derives both global and local error estimates ( Supplementary Fig. 7 ). The models reached absolute QMEAN standard scores ( Z -scores) [54] of −1.20 and −1.15 for DOT1A and DOT1B, respectively, which are in the range of the average Z -score obtained for experimentally determined structures by NMR spectroscopy [54] . All figures containing molecular structures were generated with UCSF Chimera [55] . Statistical analysis Student’s t -test was used for two-group comparisons. * P -value <0.05, ** P -value <0.01 and *** P -value <0.001 were considered significant. How to cite this article : Dindar, G. et al. Structure-guided mutational analysis reveals the functional requirements for product specificity of DOT1 enzymes. Nat. Commun. 5:5313 doi: 10.1038/ncomms6313 (2014).